Massive parallel sequencing uncovers actionableFGFR2–PPHLN1fusion andARAFmutations in intrahepatic cholangiocarcinoma Intrahepatic cholangiocarcinoma (iCCA) is a fatal bile duct cancer with dismal prognosis and limited therapeutic options. By performing RNA- and exome-sequencing analyses, we report a novel fusion event, FGFR2–PPHLN1 (16%), and damaging mutations in the ARAF oncogene (11%). Here we demonstrate that the chromosomal translocation t(10;12)(q26;q12) leading to FGFR2–PPHLN1 fusion possesses transforming and oncogenic activity, which is successfully inhibited by a selective FGFR2 inhibitor in vitro . Among the ARAF mutations, N217I and G322S lead to activation of the pathway and N217I shows oncogenic potential in vitro . Screening of a cohort of 107 iCCA patients reveals that FGFR2 fusions represent the most recurrent targetable alteration (45%, 17/107), while they are rarely present in other primary liver tumours (0/100 of hepatocellular carcinoma (HCC); 1/21 of mixed iCCA-HCC). Taken together, around 70% of iCCA patients harbour at least one actionable molecular alteration ( FGFR2 fusions, IDH1/2 , ARAF , KRAS , BRAF and FGF19 ) that is amenable for therapeutic targeting. Intrahepatic cholangiocarcinoma (iCCA) is an aggressive malignancy with a 5-year survival rate less than 10% (ref. 1 ). Surgery is the only curative option for iCCA, although it is limited to patients with early-stage disease [2] . The majority of iCCA patients are diagnosed at more advanced stages, where there is no accepted standard of care [2] , [3] . Therefore, there is an unmet need to develop a first-line therapy for these patients [2] . A deeper knowledge of the molecular mechanisms underlying this disease is crucial for the development of new effective targeted therapies. Of late, there has been a significant improvement in our understanding of the molecular basis of iCCA [4] . Large-scale molecular profiling studies have enabled the first molecular classifications to emerge [5] , [6] . Furthermore, deep-sequencing studies have provided a preliminary description of somatic mutations for iCCA [7] , [8] , [9] , [10] : novel mutations in chromatin remodelling genes ( BAP1 , ARID1A and PBRM1 ) have been recently unveiled, whereas frequent mutations in KRAS , IDH1 and IDH2 have been confirmed [8] , [9] , [10] , [11] . Nonetheless, none of the targetable mutations have been explored yet in early clinical trials. In addition to somatic mutations, somatic gene fusions are able to drive the development of human cancers, though their translational relevance has been mostly limited to haematological malignancies [12] . The recent discovery of novel fusion events associated with different types of solid tumours, such as prostate [13] , lung [14] and breast [15] cancer has increased the interest in these genetic alterations. In fact, one of such fusions (the EML–ALK fusion in lung cancer) has emerged as a druggable target and its inhibition leads to survival improvements [16] . Interestingly, a variety of FGFR2 gene fusions have been recently identified in iCCA [17] , [18] , [19] , [20] , suggesting that these events may represent novel candidate therapeutic targets and that similar strategies could be used for its clinical management. Massive parallel sequencing technology allows the characterization of cellular transcriptomes and genomes at single-base resolution, including the detection of somatic gene mutations and intragenic fusions that may lead to oncogenic molecular pathway activation. To uncover candidate oncogenes that may represent novel targets for iCCA therapy, we profile a cohort of 122 iCCA cases by performing RNA and DNA sequencing (discovery set: seven and eight paired iCCA samples analysed, respectively; screening cohort: 114 iCCA tissues). We discover a novel recurrent oncogenic fusion gene, FGFR2 – PPHLN1 (16%) and damaging mutations in the oncogene ARAF (11%). The screening of a large iCCA cohort reveals that around 70% of the tumours harbour at least one targetable molecular alteration (for example, FGFR2 fusions, KRAS/BRAF/EGFR/IDH mutations) with ~45% of patients analysed positive for at least one FGFR2 rearrangement. Significantly, the transforming and oncogenic activity of the FGFR2–PPHLN1 fusion can be successfully inhibited by a selective FGFR2 inhibitor (BGJ398) in vitro . Together our work unveils a large fraction of iCCA patients with specific targetable molecular alterations and reveals FGFR2 rearrangements as the most recurrent molecular alteration event reported so far in this disease. Identification of a novel FGFR2 fusion event in iCCA We performed single-end RNA sequencing (RNA-seq) using high-quality complementary DNA (cDNA) from seven tumour and adjacent non-tumour liver tissues of resected human iCCA. 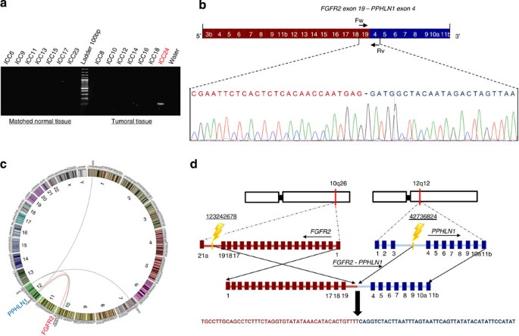Figure 1: Transcriptome analysis identified a novelFGFR2–PPHLN1fusion event. (a) RT–PCR of all seven paired tumour/normal cases using primers spanning the breakpoint confirmed the presence of a band only in the index case and not in its normal counterpart. (b) Schematic representation of the identified mRNA fusion gene.FGFR2–PPHLN1fusion mRNA is represented. Sanger sequencing confirmed the chimeric junction betweenFGFR2andPPHLN1(arrows indicate the position of the primers used for RT–PCR and Sanger sequencing). (c)FGFR2andPPHLN1genes map to 10q26 and 12q12, respectively. These genes are normally transcribed in opposite directions. WGS of the tumoral case and matched normal tissue where theFGFR2fusion was identified confirmed the presence of a translocation t(10;12)(q26;q12) as responsible mechanism for the generation of the chimeric fusion gene. Circle plot for this translocation is represented. (d) Schematic representation of the translocation responsible for the generation of aFGFR2–PPHLN1in frame event. PCR on the DNA and subsequent Sanger sequencing confirmed the exact breakpoint in the intron 20 and 3 ofFGFR2andPPHLN1, respectively. Schematic representation of the sequence around the breakpoint is here reported. By applying stringent statistical criteria across the different steps of a robust fusion identification pipeline (see detailed online methods), we identified a total of 13 novel inter- and intrachromosomal fusion events ( Supplementary Table 1 ). The best supported (top ranked) fusion event was an interchromosomal fusion comprising a portion of the tyrosine kinase receptor FGFR2 with PPHLN1 , a gene involved in epithelial differentiation. The FGFR2–PPHLN1 was represented by 149 split reads harbouring the fusion junction of exon 19 of FGFR2 to exon 4 of PPHLN1 ( Supplementary Table 1 ) and was identified in one out of the seven patients analysed (14.3%). Using primers spanning the breakpoint, we confirmed the fusion in the discovery tumour case by reverse transcriptase-PCR (RT–PCR) and subsequent Sanger sequencing of the PCR product ( Fig. 1a,b ). We then characterized the complete sequence of the 5′ FGFR2 fused to the 3′ PPHLN1 by performing broad-range PCR using primers spanning the starting codon of FGFR2 and the 3′untranslated region of PPHLN1 ( Supplementary Fig. 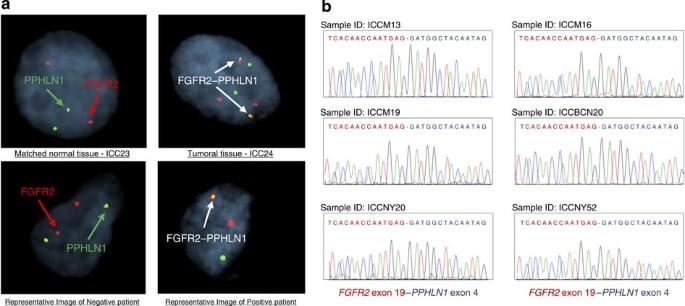Figure 2: Incidence ofFGFR2–PPHLN1and FISH validation. (a) FISH confirmed the co-localization ofFGFR2andPPHLN1probes in the tumour of the case where it was identified but not in its normal tissue [upper panel: (left) representative image of the non-tumoral tissue ICC23, arrows indicate normal, fusion-negative alleles; (right) representative image of the tumoral tissue ICC24 positive for theFGFR2rearrangement. White arrows indicate theFGFR2–PPHLN1translocation]. To determine the incidence of this fusion event in iCCAs, we screened a cohort of 107 FFPE tumours. FISH was used to confirm the presence of DNA rearrangement in 10 FFPE cases (four positive and six negative) previously screened by RT–PCR and Sanger sequencing [lower panel: (left) representative FISH image of a negative patient; (right) representative FISH detection ofFGFR2–PPHLN1in a positive patient; white arrows indicate the translocation]. Results were concordant in all but one case where the patient was called positive by FISH but not by RT–PCR screening revealing 90% concordance between the two techniques. This discrepancy might suggest a higher sensitivity of FISH over RT–PCR in this particular case probably due to the high texture admixture observed in this sample. (b) RT–PCR and subsequent Sanger sequencing identified the exact fusion breakpoint in 16% of patients (17/107). Sanger sequencing of six representative patients is shown herein. 1a , Supplementary Table 2 ). We verified that the first 19 exons of FGFR2 were present at the 5′ end of the fusion gene with an intact open reading frame and kinase domains, suggesting its preserved kinase activity. At the 3′ end, the fusion partner PPHLN1 was missing only the first three exons of which the first two are usually untranslated. Both partners have been reported to exhibit tissue-specific splicing [21] . RNA-seq data of the fusion case revealed that FGFR2IIIb isoform (Genbank accession number NM-022970 ) and PPHLN1 isoform 3 (accession number NM_201439.1 ) were the most abundant transcripts involved in the fusion protein ( Supplementary Fig. 1b ). Figure 1: Transcriptome analysis identified a novel FGFR2–PPHLN1 fusion event. ( a ) RT–PCR of all seven paired tumour/normal cases using primers spanning the breakpoint confirmed the presence of a band only in the index case and not in its normal counterpart. ( b ) Schematic representation of the identified mRNA fusion gene. FGFR2–PPHLN1 fusion mRNA is represented. Sanger sequencing confirmed the chimeric junction between FGFR2 and PPHLN1 (arrows indicate the position of the primers used for RT–PCR and Sanger sequencing). ( c ) FGFR2 and PPHLN1 genes map to 10q26 and 12q12, respectively. These genes are normally transcribed in opposite directions. WGS of the tumoral case and matched normal tissue where the FGFR2 fusion was identified confirmed the presence of a translocation t(10;12)(q26;q12) as responsible mechanism for the generation of the chimeric fusion gene. Circle plot for this translocation is represented. ( d ) Schematic representation of the translocation responsible for the generation of a FGFR2–PPHLN1 in frame event. PCR on the DNA and subsequent Sanger sequencing confirmed the exact breakpoint in the intron 20 and 3 of FGFR2 and PPHLN1 , respectively. Schematic representation of the sequence around the breakpoint is here reported. Full size image In the normal genome, FGFR2 and PPHLN1 map to chromosome 10q26 and 12q12, respectively, and are transcribed in opposite directions. To verify the presence of a genomic DNA rearrangement, we performed whole-genome sequencing (WGS) of the tumour and matched non-tumour tissue where the fusion was identified by RNA-seq. A translocation between chr10 and 12 was identified in the tumour and not in the corresponding non-tumour tissue as the mechanism responsible for the fusion gene FGFR2 – PPHLN1 ( Fig. 1c ). These data allowed us to specifically map the intronic junctions of the FGFR2–PPHLN1 fusion gene and, using specific primers and subsequent Sanger sequencing, we were able to annotate the sequence around the breakpoint ( Fig. 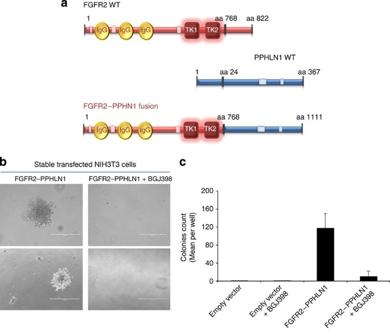Figure 3: Transforming potential of the FGFR2–PPHLN1 fusion protein. (a) Schematic representation of the fusion protein FGFR2–PPHLN1 is shown. Also normal FGFR2 and PPHLN1 protein are represented. (b) Soft agar assay for colony formation was performed with NIH3T3 cells stably transfected with V5-tagged FGFR2–PPHLN1 and empty vector. NIH3T3 cells expressingFGFR2–PPHLN1showed anchorage-independent colony formation in soft agar (left panel), which was almost completely suppressed by the addition of 1 μM of BGJ398 (P<0.001, Student’st-test, right panel). Representative images are here shown (scale bar for top panels, 400 μm, scale bar for bottom panels, 1,000 μm). (c) Quantification of colonies for NIH3T3 cells overexpressingFGFR2–PPHLN1grown with or without BGJ398. NIH3T3 cells transfected with empty vector are also indicated. Graph represents the mean±s.d. of cell counts for three separate wells of three independent experiments (mean+s.d.). 1c,d , Supplementary Table 3 ). The fusion was further confirmed by fluorescent in situ hybridization (FISH) using two specific probes for FGFR2 and PPHLN1 ( Fig. 2a , upper panel). As expected, the two probes co-localized only in the tumour tissue with the fusion transcript. Figure 2: Incidence of FGFR2–PPHLN1 and FISH validation. ( a ) FISH confirmed the co-localization of FGFR2 and PPHLN1 probes in the tumour of the case where it was identified but not in its normal tissue [upper panel: (left) representative image of the non-tumoral tissue ICC23, arrows indicate normal, fusion-negative alleles; (right) representative image of the tumoral tissue ICC24 positive for the FGFR2 rearrangement. White arrows indicate the FGFR2–PPHLN1 translocation]. To determine the incidence of this fusion event in iCCAs, we screened a cohort of 107 FFPE tumours. FISH was used to confirm the presence of DNA rearrangement in 10 FFPE cases (four positive and six negative) previously screened by RT–PCR and Sanger sequencing [lower panel: (left) representative FISH image of a negative patient; (right) representative FISH detection of FGFR2–PPHLN1 in a positive patient; white arrows indicate the translocation]. Results were concordant in all but one case where the patient was called positive by FISH but not by RT–PCR screening revealing 90% concordance between the two techniques. This discrepancy might suggest a higher sensitivity of FISH over RT–PCR in this particular case probably due to the high texture admixture observed in this sample. ( b ) RT–PCR and subsequent Sanger sequencing identified the exact fusion breakpoint in 16% of patients (17/107). Sanger sequencing of six representative patients is shown herein. Full size image To determine if this fusion gene is a recurrent event in iCCA tumours, we screened 107 formalin-fixed cases of iCCA by RT–PCR and Sanger sequencing (screening cohort). Seventeen cases (16%) were found positive for the presence of the fusion. In all positive cases, the mRNA sequence around the breakpoint was identical to the initial fusion ( Fig. 2b ). We then explored the fusion event by using FISH in 10 cases of our screening cohort (six negative and four positive patients) and obtained 90% concordance between FISH and RT–PCR screening results ( Fig. 2a , lower panel). Together our screening identified a novel FGFR2 fusion in iCCA, which accounts for 16% of the cohort here analysed. Transforming potential of FGFR2–PPHLN1 FGFR fusion events have been recently identified in several cancers. Multiple partners have been discovered including BICC1 , AFF3 , CASP7 and CCDC6 among others [17] , [18] , [19] , [20] . These different partners play an important role in the control of enforced oligomerization and subsequent trans -autophosphorylation and activation of the tyrosine kinase gene involved in the rearrangement [12] , [17] , [21] . In our case, the resulting protein ( Fig. 3a ) was predicted to contain 1111 amino acids (122 kDa) with the amino-terminal portion (residues 1–768) identical to that of FGFR2, whereas the carboxy-terminal portion (residues 769–1,111) was identical to PPHLN1 starting at residue 25 of the wild-type (WT) protein ( Supplementary Fig. 1c ). Interestingly, the C terminus domain of the WT PPHLN1 protein could be responsible for homodimerization [22] . To verify if PPHLN1 is able to mediate dimerization and activation of the FGFR2 in the fusion gene, we expressed V5-tagged FGFR2 – PPHLN1 in 293T cells and performed immunoprecipitation ( Supplementary Fig. 2a ). We successfully demonstrated constitutive activation of the fusion protein as indicated by the increased level of tyrosine phosphorylation of the fusion kinase compared with the FGFR2 WT ( Supplementary Fig. 2b , right panel) and activation of downstream MAP kinase ERK1/2 ( Supplementary Fig. 2c ). Figure 3: Transforming potential of the FGFR2–PPHLN1 fusion protein. ( a ) Schematic representation of the fusion protein FGFR2–PPHLN1 is shown. Also normal FGFR2 and PPHLN1 protein are represented. ( b ) Soft agar assay for colony formation was performed with NIH3T3 cells stably transfected with V5-tagged FGFR2–PPHLN1 and empty vector. NIH3T3 cells expressing FGFR2–PPHLN1 showed anchorage-independent colony formation in soft agar (left panel), which was almost completely suppressed by the addition of 1 μM of BGJ398 ( P <0.001, Student’s t -test, right panel). Representative images are here shown (scale bar for top panels, 400 μm, scale bar for bottom panels, 1,000 μm). ( c ) Quantification of colonies for NIH3T3 cells overexpressing FGFR2–PPHLN1 grown with or without BGJ398. NIH3T3 cells transfected with empty vector are also indicated. Graph represents the mean±s.d. of cell counts for three separate wells of three independent experiments (mean+s.d.). Full size image We then assessed the transforming potential of FGFR2–PPHLN1 fusion protein reported herein. To this purpose, NIH3T3 cells were stably transfected to overexpress V5-tagged FGFR2–PPHLN1 and empty vector. As shown in Fig. 3b,c , NIH3T3 cells expressing FGFR2–PPHLN1 showed anchorage-independent colony formation in soft agar, which was completely suppressed by the addition of the selective FGFR2 inhibitor BGJ398 (1 μM) to the culture. To further characterize the functional role of the identified fusion in an iCCA in vitro model, we generated a stable HUCCT1 cell line overexpressing FGFR2–PPHLN1 . Cells harbouring the fusion presented increased viability, clonogenic and migratory capacity ( Supplementary Fig. 3a,b ), suggesting an oncogenic capability of the fusion protein. Furthermore, HUCCT1 cells overexpressing the fusion protein showed an enhanced sensitivity to BGJ398 compared with their parental cell line transfected with the empty vector ( P <0.001, Student’s t -test, Fig. 4a,b ). In particular, significant inhibition of the migratory capability was observed only in the cells expressing the fusion protein ( P <0.0001, Student’s t -test, Fig. 4b ). The above findings support the transforming and oncogenic potential of the FGFR2–PPHLN1 fusion protein and the possible efficacy of FGFR2 inhibitors in the clinical management of iCCA patients harbouring FGFR2 rearrangements. 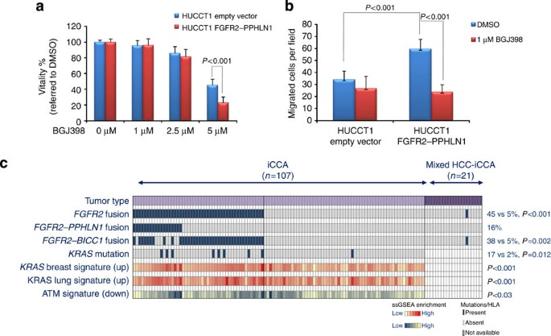Figure 4: FGFR2 fusions represent a potential therapeutic target. (a) HUCCT1 cell line transfected to overexpressFGFR2–PPHLN1showed an increased sensitivity to BGJ398 (5 μM) compared to its parental cell line transfected with the empty vector (P<0.001, Student’st-test). Reading was performed after 72 h incubation with BGJ398. Results were normalized to dimethylsulphoxide (DMSO)-treated controls and presented as the mean of three independent experiments (mean+s.d.). (b) BGJ398 (1 μM) was able to reduce cell migration only in HUCCT1 cell line expressing FGFR2–PPHLN1 (P<0.0001, Student’st-test). (c) A validation cohort of 107 iCCAs was screened for the presence of FGFR2 fusions.FGFR2–PPHLN1and the previously reportedFGFR2–BICC1were present in 16% and 38% of iCCA cases, respectively, and were not mutually exclusive. Presence ofFGFR2rearrangements was also investigated in 21 mixed HCC–iCCA tumours (here shown) and 100 HCCs. Only one mixed HCC–iCCA tumour belonging to the histological subtype of stem cell features was found positive forFGFR2–BICC1. NoFGFR2fusion was identified in any of the HCC samples analysed. Significant association was found between presence ofFGFR2fusion and KRAS pathway activation in breast and lung (P<0.001, Student’st-test) and/orKRASactivating mutation (P=0.01, Fisher’s exact test). Significant ATM target downregulation was observed in patients harbouringFGFR2rearrangements. Enrichment scores for each sample were calculated by ssGSEA and is displayed here as a heatmap. Figure 4: FGFR2 fusions represent a potential therapeutic target. ( a ) HUCCT1 cell line transfected to overexpress FGFR2–PPHLN1 showed an increased sensitivity to BGJ398 (5 μM) compared to its parental cell line transfected with the empty vector ( P <0.001, Student’s t -test). Reading was performed after 72 h incubation with BGJ398. Results were normalized to dimethylsulphoxide (DMSO)-treated controls and presented as the mean of three independent experiments (mean+s.d.). ( b ) BGJ398 (1 μM) was able to reduce cell migration only in HUCCT1 cell line expressing FGFR2–PPHLN1 ( P <0.0001, Student’s t -test). ( c ) A validation cohort of 107 iCCAs was screened for the presence of FGFR2 fusions. FGFR2–PPHLN1 and the previously reported FGFR2–BICC1 were present in 16% and 38% of iCCA cases, respectively, and were not mutually exclusive. Presence of FGFR2 rearrangements was also investigated in 21 mixed HCC–iCCA tumours (here shown) and 100 HCCs. Only one mixed HCC–iCCA tumour belonging to the histological subtype of stem cell features was found positive for FGFR2–BICC1 . No FGFR2 fusion was identified in any of the HCC samples analysed. Significant association was found between presence of FGFR2 fusion and KRAS pathway activation in breast and lung ( P <0.001, Student’s t -test) and/or KRAS activating mutation ( P =0.01, Fisher’s exact test). Significant ATM target downregulation was observed in patients harbouring FGFR2 rearrangements. Enrichment scores for each sample were calculated by ssGSEA and is displayed here as a heatmap. Full size image FGFR2 fusions are the most recurrent molecular alterations To elucidate the prevalence of FGFR2 fusion events in iCCA, we also screened our large iCCA cohort (screening set) for the presence of the FGFR2–BICC1 fusion [17] . This screening revealed that 38% (40/107) of the analysed tumours harboured the FGFR2–BICC1 fusion transcript ( Fig. 4c ). Interestingly, FGFR2 fusions ( FGFR2–PPHLN1 and FGFR2–BICC1 ) were not mutually exclusive and overall 45% of iCCA patients (48/107) harboured at least one FGFR2 fusion. FGFR2 fusions were not detected in a set of 100 hepatocellular carcinomas (HCCs) and were very rare in mixed HCC–iCCA cancers, with only one case out of 21 patients analysed (5%) harbouring a FGFR2–BICC1 fusion gene ( Fig. 4c ). No significant association of the FGFR2 fusions was found with clinico-pathological parameters or outcome ( Supplementary Table 4 ). Single-sample gene set enrichment analysis (ssGSEA) in genome-wide transcriptome profiles of 107 tumours of the screening set revealed a significant enrichment of genes in the KRAS signalling pathway in the tumours harbouring the FGFR2 fusions ( P <0.001, Student’s t -test, Fig. 4c ). When we performed classic GSEA comparing the patients with FGFR2 fusions versus the rest, KRAS pathways were found among the top enriched ones ( P <0.05, false discovery rate (FDR)<0.05, Kolmogorov–Smirnov statistic test). Consistently, 90% of the patients harbouring KRAS mutations were also positive for FGFR2 fusions, suggesting cooperation between these two pathways ( Fig. 4c , P =0.01, Fisher’s exact test). FGFR2 is located within the Aphidicolin-inducible fragile site FRA10F on chr10q26.1 (ref. 23 ). Several DNA-damage response proteins have been shown to regulate the stability of fragile sites [24] , [25] , including Ataxia telangiectasia mutated (ATM) and Rad3 related (ATR) and its effector Chk1 (ref. 26 ). Interestingly, ATM pathway genes were found to be significantly downregulated in patients harbouring FGFR2 fusions as revealed by ssGSEA ( Fig. 4c , P <0.03, Fisher’s exact test) and by classic GSEA ( P <0.05, FDR<0.05, Kolmogorov–Smirnov statistic test). These observations imply that FGFR2 rearrangements represent the most recurrent molecular alteration event reported so far in iCCA. Furthermore, frequent co-occurrence of KRAS mutations and FGFR2 fusion events suggests a possible cooperative role in driving iCCA pathogenesis, whereas the deregulation of pathways involved in the stability of fragile sites may be responsible for the occurrence of such rearrangements. Exome sequencing identifies novel ARAF mutations We explored exome sequencing (exome-seq) data generated on eight pairs of iCCA tumour and paired non-tumour tissues (seven equal cases as above). We identified 237 alterations in the coding regions including 229 mutations affecting 209 genes (range 18–53, average 30 per tumour) and eight insertions and deletions (indels; Supplementary Fig. 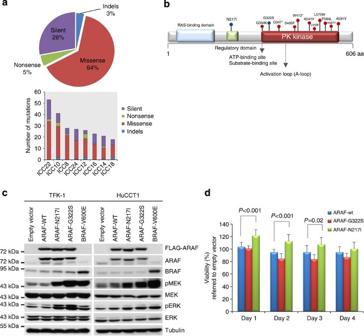Figure 5: Mutational landscape of iCCA. (a) Pie chart representation of non-synonymous somatic mutations (upper panel) and number of non-synonymous somatic mutations per sample across eight iCCA cases (lower panel). (b) Schematic representation of theARAFgene and exact location of the identified mutations, including the two found by exome-seq (blue) or by Sanger sequencing (red). (c) Western blot images of TFK-1 and HuCCT1 cell line transfected withARAFWT,ARAFN217I, G322S and BRAF V600E as control for downstream activation. Images show an increased phosphorylation of MEK and ERK in cells transfected with mutatedARAF, similar to the cells overexpressingBRAF V600E. (d) MTS assay of the TFK-1 cell line transfected to express empty vector, WTARAFand mutantARAF. Cell lines expressing N217IARAFmutant showed an increased viability compared with the parental cell line. Readings were performed after 24 h (day 1), 48 h (day 2), 72 h (day 3) and 96 h (day 4). Results were normalized to the empty vector-transfected control and presented as the mean of three independent experiments (mean+s.d.). 4 , Supplementary Table 5 ). Somatic substitutions were predominantly C:G>T:A transitions as previously reported in iCCA and other cancers [7] , [8] , [9] , [10] , [11] . Of the mutations identified, 64% were missense, 28% were silent, 5% were nonsense and 3% were indels ( Fig. 5a ). 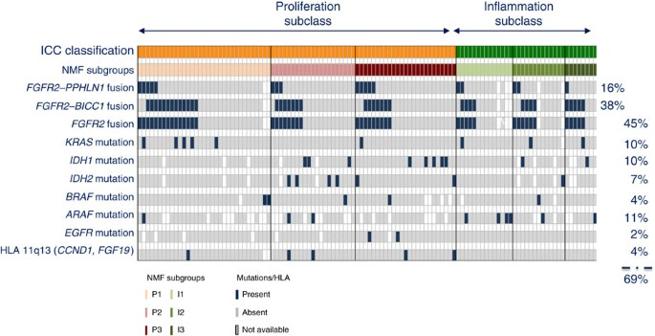Figure 6: About 70% of iCCA patients harbour at least one targetable molecular alteration. Image shows the integration of our previously published molecular classification5with the results of the mutational and fusion events screened in 114 iCCAs. TheFGFR2fusion discovered here,FGFR2–PPHLN1, and the previously reportedFGFR2–BICC1, were identified in 16% and 38% of the cohort, respectively. The twoFGFR2fusions were found to be not mutually exclusive, with 45% of patients analysed harbouring at least oneFGFR2event. The presence of specific hot-spot mutations was investigated in the cohort and is reported here (blue, present; grey, absent; white, not available). In brief,KRASandIDH1/2mutations were found in 10 and 17%, respectively, of patients analysed.ARAFwas mutated in 11%,BRAFin 4%,EGFRin 2% and high-level amplification 11q13 in 4% of the patients analysed. Overall, 69% (79/114) of the entire cohort harboured at least one targetable molecular alteration. Globally, 199 genes were mutated in only one patient, nine genes were mutated in two patients ( Supplementary Table 6 ) and 13 genes presented more than one mutation ( Supplementary Table 7 ). Among the 163 non-synonymous mutations identified, 75 were predicted to have damaging functional consequences by using the Polyphen-2 algorithm (range 5–17, average 9 per sample, Supplementary Table 8 ), including a novel truncating mutation in ARID1A and two missense mutations in the ARAF gene, G322S, a novel mutation in the kinase domain and N217I, which has been previously reported [7] ( Supplementary Fig. 5a ). ARAF mutations were confirmed by independent PCR and sequencing in each tumour. External validation of the identified ARAF mutations along with the screening of the entire kinase domain (exons 10–16) of the gene revealed the presence of 11 different mutations in nine patients out of 84 (11%; Fig. 5b , Supplementary Table 9 ). The novel mutations included two nonsense and nine missense mutations ( Supplementary Table 9 ). All missense mutations were predicted to be damaging by Polyphen-2. To investigate whether these mutations were somatic, the surrounding non-tumoral tissue and nine non-neoplastic liver tissues were analysed by PCR and Sanger sequencing ( Supplementary Figs 6–8 ). In three patients, the non-surrounding tissue was available and the analysis confirmed that the four identified mutations (A541V, G322S, S469F and W472*) were indeed bona fide somatic ( Supplementary Figs 6,7 ). In addition, none of the nine normal livers analysed carried the mutations, thus suggesting that these mutations are more likely to represent somatic events. To verify the impact of the most frequent mutations on the activity of the protein, we overexpressed WT ARAF and N217I and G322S mutant variants in CCA cell lines (TFK-1 and HUCCT1). Western blot analysis showed increased phosphorylation of the downstream molecule MEK in cells overexpressing the N217I and G322S mutants compared with empty vector and ARAF WT ( Fig. 5c ). Furthermore, the cell lines expressing the N217I ARAF mutant showed increased viability compared with the parental cell line, whereas G322S mutant had no effect or slightly slowed cellular viability ( Fig. 5d , Supplementary Fig. 5b ). N217I and G322S mutations were not able to transform NIH3T3 in vitro suggesting that further studies need to be conducted to clarify the potential oncogenic role of these mutations in iCCA. Of note, we have demonstrated that ARAF mutations G322S and N217I are able to induce the constitutive activation of the downstream pathway and N217I might possess oncogenic activity in vitro. Furthermore, our screening identified novel damaging mutations in the ARAF oncogene, which occur in 11% of the iCCA patients. Figure 5: Mutational landscape of iCCA. ( a ) Pie chart representation of non-synonymous somatic mutations (upper panel) and number of non-synonymous somatic mutations per sample across eight iCCA cases (lower panel). ( b ) Schematic representation of the ARAF gene and exact location of the identified mutations, including the two found by exome-seq (blue) or by Sanger sequencing (red). ( c ) Western blot images of TFK-1 and HuCCT1 cell line transfected with ARAF WT, ARAF N217I, G322S and BRAF V600E as control for downstream activation. Images show an increased phosphorylation of MEK and ERK in cells transfected with mutated ARAF , similar to the cells overexpressing BRAF V600E . ( d ) MTS assay of the TFK-1 cell line transfected to express empty vector, WT ARAF and mutant ARAF . Cell lines expressing N217I ARAF mutant showed an increased viability compared with the parental cell line. Readings were performed after 24 h (day 1), 48 h (day 2), 72 h (day 3) and 96 h (day 4). Results were normalized to the empty vector-transfected control and presented as the mean of three independent experiments (mean+s.d.). Full size image Integrative analysis unveils specific iCCA subgroups To provide an overview of the genomic landscape of molecular alterations in iCCA, we integrated exome- and RNA-seq data with our previously published iCCA molecular classification [5] . IDH1 and IDH2 mutations were observed in 11 (11/107, 10%) and 7 patients, respectively (7/107, 7%, Supplementary Table 10 ). Interestingly, patients with IDH1 and IDH2 mutations were significantly enriched in P2–P3 subgroups of our proliferation subclass (15/45 versus 3/62 rest, P <0.001, Fisher’s exact test, Fig. 6 ), which is associated with chromosomal instability, enrichment of a stem cell-like iCCA signature [27] and activation of EGFR signalling. Consistent with the functions of IDH1/2 enzymes, the pathways related to tricarboxylic acid cycle and electron transport were enriched in patients with IDH mutations (FDR<0.05, Supplementary Table 11 ). Moreover, a recently published iCCA signature with stem cell-like features [27] was significantly enriched in IDH mutant tumours [28] along with several oncogenic pathways including KRAS , MET , NOTCH and VEGF pathways. Figure 6: About 70% of iCCA patients harbour at least one targetable molecular alteration. Image shows the integration of our previously published molecular classification [5] with the results of the mutational and fusion events screened in 114 iCCAs. The FGFR2 fusion discovered here, FGFR2–PPHLN1 , and the previously reported FGFR2–BICC1 , were identified in 16% and 38% of the cohort, respectively. The two FGFR2 fusions were found to be not mutually exclusive, with 45% of patients analysed harbouring at least one FGFR2 event. The presence of specific hot-spot mutations was investigated in the cohort and is reported here (blue, present; grey, absent; white, not available). In brief, KRAS and IDH1/2 mutations were found in 10 and 17%, respectively, of patients analysed. ARAF was mutated in 11%, BRAF in 4%, EGFR in 2% and high-level amplification 11q13 in 4% of the patients analysed. Overall, 69% (79/114) of the entire cohort harboured at least one targetable molecular alteration. Full size image iCCA tumours harbouring the FGFR2 fusions did not show significant enrichment in any of the iCCA subclasses ( Fig. 6 ). As above described, there was a significant association between the presence of FGFR2 fusions and KRAS activating mutations ( P =0.01, Fisher’s exact test). No significant association was found with other mutations analysed such as ARAF (11%), BRAF (4%), IDH1/2 (17%), EGFR (2%) and high-level amplification at 11q13 (4%) ( Fig. 6 ) [5] . Overall, 69% (79/114) of iCCA patients harboured at least one targetable molecular alteration ( Fig. 6 ) and more likely may respond to targeted molecular therapies highlighting the relevance of translating these findings to clinical settings. iCCA is an orphan disease for which there is currently no first-line approved standard of care for unresectable cases [2] . Here we provide compelling evidence indicating that FGFR2 fusions, including the novel FGFR2–PPHLN1 fusion, are highly frequent molecular aberrations in iCCA (~45%) and might represent a therapeutic opportunity. In addition to the detection of these fusion events, we describe previously unknown damaging mutations in the ARAF oncogene (11%) and define a complete landscape of targetable mutations in this cancer (for example, IDH1/2 , BRAF , KRAS , EGFR ) occurring in at least 70% of patients. The identification of the EML4–ALK fusion in a small subgroup of patients with lung cancer has provided the rationale for demonstrating survival benefits for specific molecular therapies, such as crizotinib [16] . The short time frame elapsed between the discovery of the fusion [14] , the conduction of a proof-of-concept trial [29] and the final demonstration of survival benefits, have opened a new paradigm for translating oncodriver discoveries into clinical practice. Our current study provides a comprehensive landscape of molecular alterations occurring in iCCA and unveils a surprising high prevalence of FGFR2 fusions, which are therefore expected to have clinical impact as therapeutic targets. Our functional analysis demonstrated that the newly identified FGFR2–PPHLN1 fusion possesses transforming and oncogenic capability and can be effectively targeted by a small-molecule FGFR2 inhibitor. In our study, FGFR2 fusions were found in 45% of iCCA patients, in 5% of HCC–iCCA mixed tumours and were absent in HCC. These data are consistent with recent reports where FGFR2 fusions were reported in iCCA (9/66, 14%) but rarely in HCC (1/98) (ref. 19 ). Nonetheless, the incidence of FGFR2 fusions strikingly differs across the iCCA published cohorts, with a range between 50% in small series [17] , [18] to 10–15% in series of up to 96 patients [19] , [20] , [30] . Overall, our cohort consisted of Caucasian patients at early-intermediate stage iCCA amenable for resection, whereas other series mostly refer to Asian patients at more advanced stage of disease [19] . In our study, no differences in terms of gender, age, viral infection, stage and prognosis was observed between patients harbouring or not FGFR2 fusions. In a Japanese study, there was a significant association between patients with viral infections and FGFR fusions, a fact not observed in our cohort [19] . Thus, while we cannot conclude from these data whether viral infections or underlying liver disease might contribute to the occurrence of FGFR2 translocations in iCCA patients, we could speculate that different ethnicity and geographical population might partially explain such discrepancy. Ad hoc larger studies need to be conducted to clarify such discrepancies. In addition, we observed that FGFR2 fusions were not mutually exclusive with each other, with 10% of the iCCA patients showing presence of both FGFR2–PPHLN1 and FGFR2–BICC1 fusion genes. There are several potential explanations for the specific presence of FGFR2 fusions in iCCA and the co-occurrence of multiple types of FGFR2 fusions in the same tumour, although it needs to be determined whether the different fusions co-exist in the same iCCA cell or represent different iCCA cells in single cell-level analysis. The presence of fragile sites and/or hot spots for genomic DNA rearrangements within the FGFR2 gene, for example, FRA10F (ref. 23 ), may explain this phenomenon. Recent studies have revealed that the presence of AT-rich sequences in the region can form highly stable secondary structures promoting DNA breakage [24] , [25] . Of note, the ATM pathway—involved in the regulation of fragile sites [26] —was found to be significantly downregulated in our patients harbouring FGFR2 rearrangements, suggesting this pathway may play an important role in the occurrence of these fusion events in iCCA. We also provided evidence that a FISH-based assay can be used as a biomarker that correlates with the presence of the discovered fusion. To date, no mutations or focal amplifications have been described for FGFR2 and the reported fusions [17] , [18] , [19] , [20] appear to be the main mechanism of activation of this oncogene and could be explored for trial enrichment. For example, early clinical trials exploring the concept of potential oncogenic addiction to FGFR2 could be enriched by iCCA patients with positive FGFR2 fusions detected by FISH. Nonetheless, although tumour tissue-based FISH is a clinically applicable measure to detect the presence of FGFR2 fusions [18] , [19] , [30] , their detection in plasma or serum may enable less invasive and more flexible screening strategies that potentially provide indication for FGFR2 inhibitors in treating advanced-stage iCCAs. In this sense, studies correlating liquid biopsy findings with iCCA tissue FGFR2 fusions are expected. FGFR2 fusions were not mutually exclusive with the presence of other mutations. Activating mutations of KRAS are frequent molecular alterations in iCCA (22%, range 5–57%) [4] , as also seen in our study (10%). Interestingly, KRAS mutation-positive tumours also harbour the FGFR2 fusions (90%), suggesting their cooperative role in driving iCCA pathogenesis. This association was not observed in a previous genomic study of iCCA [19] and thus the finding needs to be further confirmed. A handful of mutations identified so far in iCCA can be potentially targeted by specific drugs. Novel mutations in chromatin remodelling genes (for example, ARID1A , BAP1 and PBMR1 ) have emerged and account for the most frequent mutations reported so far in iCCA (~25%) [8] , [9] as it has also been corroborated in recent studies where mutations in such genes have been identified even at higher frequency (34–46%) [10] , [20] . At the same time, already described mutations (for example, KRAS , IDH1/2 , and EGFR ) have been confirmed [7] , [8] , [9] , [10] , [11] , [20] . Notably, IDH1/2 -activating mutations occur in ~20% of the iCCA cases [4] —17% in our series—and tend to be mutually exclusive with other mutations. Phase I trials with specific inhibitor of IDH1/2 mutations are currently ongoing in cholangiocarcinoma patients. In the current study, by applying exome-seq and screening of a large cohort, we confirmed some known mutations (for example, ARID1A , IDH1/2 ) and identified two activating mutations and 10 potentially damaging mutations in ARAF , a member of the RAF oncoproteins. ARAF is a serine–threonine-specific protein kinase that activates the MEK/ERK signalling cascade downstream of RAS (ref. 31 ). ARAF mutations are rare compared to BRAF and CRAF (ref. 32 ). In this study, we identified two mutations in ARAF : N217I, which had been previously reported in iCCA [7] and G322S, a novel mutation in the kinase domain. ARAF shows 90% homology with the other 2 RAF genes of the family and share three highly conserved regions (CR1–CR3) [33] . CR1, at the N terminus, is composed of a RAS-binding domain. CR2 is a regulatory region with a serine/threonine-rich domain and is followed by the protein kinase domain (CR3) near the C terminus. The ability of RAF proteins to bind to RAS is regulated by several adaptor and scaffold signalling proteins, such as 14-3-3 proteins. The N217I mutation is located in the regulatory region close to one of the known sites of phosphorylation and 14-3-3 binding (S214). Substitution of serine 214 by alanine (S214A) leads to an increased basal and inducible ARAF kinase activity when compared to the WT enzyme [34] . Similar results were also obtained with the homologous serine in BRAF (S365) indicating that the phosphorylation of this site and its interaction with 14-3-3 protein acts as a negative regulator of RAF activity [35] . The domain where G322S is located is highly conserved across all the three genes and the corresponding mutation in BRAF has been demonstrated to be activating [36] . Here we demonstrated that the mutations N217I and G322s are able to increase the phosphorylation of the downstream effectors and N217I might possess oncogenic activity in vitro. Screening of our prevalence cohort for these two mutations along with the evaluation of the kinase domain revealed that overall 11% of the iCCA population harbours mutations in ARAF gene. These mutations are novel [7] , [8] , [9] , [10] , [20] , and their oncogenic potential needs to be properly investigated in experimental models. In conclusion, we have shown that FGFR2 fusions are the most recurrent targetable molecular alteration described so far in iCCA (~50%), including the novel FGFR2–PPHLN1 fusion unveiled here by RNA-seq in 16% of the patients analysed. In addition, we identified novel mutations in the oncogene ARAF , which might represent a novel potential target, and warrants further clinical evaluation. Tumour samples and nucleic acid extraction Fresh frozen tumour tissues and corresponding normal tissue ( n =7 pairs) from resected iCCA patients were collected from the Biorepository Tissue Bank at the Icahn School of Medicine at Mount Sinai (New York) after approval by the institutional review board (IRB) committee. Informed consent was obtained for all the subjects. The samples chosen contained only tumoral tissue and were free of non-tumoral liver parenchyma. Furthermore, the diagnosis of iCCA was confirmed by an expert liver pathologist. Total RNA was extracted from homogenized iCCA samples and their normal conterparts using TRizol Regent (Invitrogen). Quantity of RNA was measured using Quant-iT Ribogreen RNA assay kit. One μg of RNA was used for subsequent RNA-seq library generation. DNA was isolated using the ChargeSwitch gDNA Mini Tissue Ki/t (Invitrogen) after tissue disruption with a homogenizer. DNA quantity was assessed through Quant-It PicoGreen dsDNA Assay kit (Invitrogen). A total of 107 formalin-fixed, paraffin-embedded (FFPE) samples were obtained from iCCA patients resected between 1995 and 2007 at three centres from the HCC Genomic Consortium: IRCCS Istituto Nazionale Tumori (Milan), Mount Sinai School of Medicine (New York) and Hospital Clinic (Barcelona). The study protocol was approved at each center’s IRB. The iCCA samples used represent a subgroup of a larger cohort ( n =149) previously published elsewhere [5] . Gene expression data of these samples has been deposited in the GEO database (GSE33327), whereas description of the entire cohort is available in Table 1 of ref. 5 . Description of the samples used in the current study is summarized in Supplementary Table 4 . Clinicopathological characteristics and follow-up data were available for 98/107 patients analysed for FGFR2 fusions (see details in Supplementary Table 4 ). A total of 21 FFPE mixed HCC–iCCA tumours were collected at the Icahn school of Medicine at Mount Sinai (New York, NY) after approval by the IRB committee. According to the WHO Classification 2010 (ref. 37 ), four cases belong to the classical type with areas of typical HCC and areas of typical CCA, whereas 17 cases belong to the stem cell type. Furthermore, 6/17 stem cell type tumours were categorized as cholangiolocellular subtype. All the tissue sections were macrodissected to avoid contamination of non-cancerous liver tissue on RNA extraction. In brief, for each classical type, the HCC part was separated from the iCCA component. Surrounding non-tumoral tissue was also extracted. For the stem cell features types, tumour was separated from the surrounding tissue but, considering the complexity of this subtype and the lack of specific markers, no further microdissection was performed for the purpose of the current study. All the different areas macrodissected were screened for the presence of FGFR2 rearrangements. Total RNA was isolated from three freshly cut 5-μm-thick FFPE sections using QIAcube (QIagen, Düsseldorf, Germany) [5] . RNA quantity was assessed using Quant-iT Ribogreen RNA assay kit (Invitrogen). A total of 100 surgically resected fresh frozen HCC samples were obtained from two institutions of the HCC Genomic Consortium: IRCCS Istituto Nazionale Tumori (Milan, Italy) and Hospital Clínic (Barcelona, Spain) after approval by the IRB committee. Tissue was pulverized using the BioPulverizor (Biospec, Bartlesville, OK) to ensure a homogenous mix of cells and stored at −80 °C. RNA was extracted using the RNeasy mini kit (Qiagen, Germantown, MD). RNA-seq technology and fusion gene identification The sequencing library was prepared with the standard TruSeq RNA Sample Prep Kit v2 protocol (Illumina, CA, USA). In brief, total RNA was poly-A-selected and then fragmented. The cDNA was synthesized using random hexamers, end-repaired and ligated with appropriate adaptors for sequencing. The library then underwent size selection and purification using AMPure XP beads (Beckman Coulter, CA, USA). The appropriate Illumina recommended 6-bp bar-code bases are introduced at one end of the adaptors during PCR amplification step. The size and concentration of the RNA-seq libraries was measured by Bioanalyzer and Qubit fluorometry (Life Technologies, USA) before loading onto the sequencer. The mRNA libraries were sequenced on the Illumina HiSeq 2500 System with 100 nucleotide single-end reads, according to the standard manufacturer's protocol (Illumina, USA). Between 20 and 25 million 100-bp reads were generated for each of the seven matched normal samples. Actual alignment of the raw cDNA reads was carried out by tophat-fusion [38] and de novo assembly of transcript level reads was carried out by Cufflinks [39] , [40] . In brief, tophat-fusion breaks up individual reads into 25-bp segments, which are mapped independently to the reference build hg19 via bowtie [41] . Following Edgren et al . [42] , we used the following filtration scheme to identify fusion events: (1) BLAST sequence around putative breakpoint to hg19 build to identify and remove paralogous sequences; (2) filter fusions based on the number of reads that support the putative fusion breakpoints, setting the minimum number of such spanning reads conservatively; (3) compute scores of distributions of coverage of reads around the putative breakpoints, rejecting non uniformly covered reads; (4) fusions between adjacent genes were rejected as read-through transcript events, with a minimum distance of 100 kb; (5) finally, we considered a read to support a fusion if it mapped to both sides of breakpoint by at least a minimum fusion anchor length of 25 bp, or generally about a quarter of a read length. All these parameters were essentially tuned with the constraint that the matched normal sample had no positive fusion detections. RNA-seq data of these samples has been deposited in the GEO database (GSE63420). Whole-exome sequencing and somatic mutation detection Genomic DNA was sheared using the Covaris E210 system (Covaris, Woburn, MA). Total genomic DNA library is generated following the manufacturer protocol (NEBNext DNA Library Prep Master Mix Set for Illumina, New England Biolabs, Ipswich, MA). At this point, the library is ready for WGS. For whole-exome sequencing, the WGS library then undergoes solution-based hybridization to an oligonucleotide pool designed to enrich for the whole-exome regions of interests. The library is captured by following the manufacturer protocol (SeqCap EZ Human Exome Library v3.0 User Guide, Roche NimbleGen, Madison, WI). Eight normal iCCA pairs (including the seven reported above) underwent whole-exome sequencing and one normal iCCA pair underwent WGS. The experiments achieved high quality in the metrics of high read quality, high mapping rate, low duplication rate and adequate coverage of the target regions. PCR and optical duplicates, low-quality (Q<20) and non-uniquely mapped reads were successfully removed. Remaining reads were aligned to the human genome reference 19th version using BWA [43] . Afterwards, somatic single-nucleotide variants and small indels were identified through VarScan2 (ref. 44 ). We calculated the P value using Fisher’s exact test for all putative mutation sites based on the distribution of read support for different alleles in tumour and matched normal samples. The VarScan2 software was employed in above analyses because of their desirable feature in detecting mutations in low purity or heterogeneous cancer samples. Purity information was factored in mutant allele frequency estimations. Structure variants were identified on WGS data, using CREST software (PMID: 21666668). Somatic single-nucleotide variants and indels inferred by VarScan2 software were filtered based on the following criteria: (1) Read depth ≥20 in both tumour and normal samples; (2) read support of mutant allele in tumour tissue not a result of a sequencing error (binomial test, P >0.01); (3) quality score not significantly lower than other alleles (Wilcoxon rank-sum test, P >0.01). (4) Mutant allele frequency change between tumour and adjacent normal ≥20% and Fisher’s exact test P value <0.01; (5) mutant allele not significantly enriched in repeatedly aligned reads; (6) mutant allele not significantly enriched within 10 bp of 5′ or 3′ ends of reads (Fisher’s exact test, P >0.01); (7) mutant alleles were observed in both forward and reverse strand of the tumor DNA; finally, the resulting mutations were annotated by the SNPEff pipeline, in terms of mutation location, impact on gene product and the likelihood of the mutation to be functional (SIFT and PolyPhen-2 scores). Structural variants were filtered based on the following criteria: (1) the breaking point site read depth ≥20; (2) at least observe five soft-clip reads; and (3) read supports observed in both strand. In brief, high-quality sequences based on low duplication rate (range 7–18%), high mapping rate (range 96 millions −158 millions reads; average 127 millions reads) and adequate coverage were achieved. Exome-seq data has been deposited in the GEO database (GSE63420). cDNA conversion and RT–PCR reaction One microgram of RNA was retrotranscribed into cDNA using the RNA to cDNA Ecodry Premix (Clontech) following manufacturer’s instructions. The resulting cDNA was used as template for semiquantitative PCR amplification using the primers reported in Supplementary Table 11 . To detect the presence of the fusion product, the PCR amplifications on human tissues were performed using the following protocol: 95 °C for 2 min, 40 cycles of 95 °C for 30 s, 55 °C for 30 s, 72 °C for 2 min. PCR amplifications were performed in a volume of 25 μl reaction mixture containing 1.5 mM MgCl 2 , 0.2 mM of each dNTP, 0.125 mM of each primer and 1 U of Platinum Taq DNA polymerase (Invitrogen). PCR products were purified using the Qiaquick PCR purification kit (Qiagen) and sequenced using an Applied Biosystems 3700 DNA sequencer (ABI PRISM 3730XL; Applied Biosystems). The cases analysed by PCR were considered positive only if Sanger sequencing successfully confirmed the sequence of the fusion mRNA around the breakpoint. For the amplification and subsequent cloning of the full fusion gene, 1 μg of RNA of the index case was reverse transcribed using 2 pmol of the gene specific reverse primer with Superscript III (Invitrogen) following manufacturer’s instructions with the exception that 1 h incubation was at 55 °C. 2 units of RNase H (NEB) was added to the reaction to remove complementary RNA and incubated at 37 °C for 20 min. Fluorescent in situ hybridization Commercially available satellite probes (FGFR2-RP11-62L18-orange 5-TAMRA dUTP and PPHLN1-RP11-154F20 5-Fluorescein dUTP) mapping to the corresponding regions of chr10:123,224,100-123,398,498 and chr12:42,694,068-42,878,307 respectively, were purchased from Empire Genomics LLC (Buffalo, NY). Four-micrometer sections from FFPE iCCA tissues were baked at 60 °C for at least 2 h and then deparaffinized and rinsed through water. The slides were incubated in a sodium thiocyanate solution (16 g sodium thiocyanate per 200 ml purified water) for 10 min at 80 °C and then washed in PBS. They were then incubated in 0.2% pepsin in 0.01 N HCl for 20 min at 37 °C followed by quenching in 2xPBS plus glycine. Slides were then postfixed in 4% paraformaldehyde then washed in PBS three times over 15 min and finally dehydrated. Previously denatured probes were added onto slides, which were then coverslipped and placed in a HYBrite chamber (Vysis, Abbott Molecular, Abbott Park, IL) where they were denatured for 3 min at 83 °C and hybridized overnight at 37 °C. Slides were washed in 50% Formamide in 1 × saline sodium citrate three times for 5 min at 37 °C, followed by three 5 min 1 × saline sodium citrate and three 0.1% Tween-20 4 × SCC washings at 37 °C. Slides were dehydrated and counterstained with mounting medium with DAPI (4′,6-diamidino-2-phenylindole,Vector Laboratories Inc., Burlingame, CA). Results of the hybridization were visualized with an automated Leica DM5500B fluorescence microscope and scored using the Leica Application Suite Advanced Fluorescence LAS AF software (Leica Microsystems Inc., Buffalo Gove, IL) following the next criteria: for each case, microphotographs of 10 microscopic high power fields (× 1,000, oil immersion) corresponding to iCCA tumour areas were obtained with DAPI, fluorescein isothiocyanate and Cy3 filters. Numbers of green and orange signals were counted for each DAPI-labelled nucleus (100 nuclei were scored for each sample). Presence of fusion was determined when the signals from the two probes (FGFR2 in red and PPHLN1 in green) were overlapping and a yellow signal was observed. Individual images of representative fusion-positive and fusion-negative iCCA cases were captured with a Zeiss Axio Imager Z2 microscope (Zeiss, Jena, Germany) with the same set of filters described above, using the CytoVision 7.2 software (Leica Microsystems Inc., Buffalo Gove, IL). Microarray data Gene expression data for the independent cohort ( n =107) were already available (Microarray GEO number: GSE33327) ref. 5 ). Genes, molecular pathways and gene expression signatures associated with the classes were evaluated using GSEA for Molecular Signature Database gene sets (MSigDB, www.broadinstitute.org/msigdb ). Data analysis was conducted using the GenePattern Analytical Toolkit, whereas the correlation with clinicopathological parameters was performed with SPSS software (version 18). Correlation between the presence of FGFR2 fusions and clinicopathological variables was assessed by Fisher’s exact test. Cell lines and FGFR2 inhibitor HUCCT1 (Riken Bioresource Center, Ibaraki, Japan) and TFK-1 (DSMZ) were maintained in RPMI supplemented with 10% heat-inactivated fetal bovine serum. Cells (293T) were grown in Dulbecco’s modified Eagle’s medium with 10% heat-inactivated fetal bovine serum. Cells were maintained at 37 °C in a 5% CO 2 atmosphere. The FGFR2 inhibitor, BGJ398, was purchased from SelleckBio ( http://www.selleckbio.com ) and added at the cell culture at different concentrations (range 100 nM–10 μM). Cloning strategy and stable transfection The fusion FGFR2–PPHLN1 cDNA was amplified by PCR using the Pfx platinum system from Invitrogen and the primers reported in Supplementary Table 12 ; 5 μl template was added to the reaction. The PCR amplifications were performed using the following protocol: 95 °C for 2 min, 45 cycles of 95 °C for 1 min, 52 °C for 1 min and 72 °C for 5mins. A secondary PCR was performed on 2 μl of primary PCR using primers designed with an attB overhang to amplify the fusion cDNA in frame for cloning into the Gateway system for mammalian expression (Invitrogen; primers sequence is reported in Supplementary Table 12 ). The attB PCR product was cloned first into pDONR-zeo to create an entry clone and then shuttled into the mammalian expression vector pcDNA 6.2Em/GFPBsd/V5-DEST according to manufacturer’s instructions to create pDEST-V5-FGFR2/PPHLN1. Cloning reactions were incubated overnight to achieve maximum recombination efficiency. Constructs were confirmed by Sanger sequencing. Expression constructs (pReceiver-M12 vector, OmicsLinkTM) containing WT human ARAF ORF (NM_001654.4) and mutation variants (N217I and G322S) were purchased from GeneCopoeiaTM (Rockville, USA). Six-well plates containing 2 × 10 5 HUCCT1 and TFK-1 cells were stably transfected with 2.5 μg linearized vectors using the Lipofectamine transfection system (Invitrogen) or X-treme gene DNA HP transfection reagent. Following 48 h of transfection, cells were selected with Blasticidin (10 μg ml −1 ) or Geneticin (500 μg ml −1 , G418 disulfate salt, Sigma). Validation of ARAF mutations and IDH mutations screening Validation of the two ARAF mutations identified by exome-seq and screening of the kinase domain PCR was performed using specific primers ( Supplementary Table 12 ). Each PCR reaction contained 1 × Platinum Taq DNA Polymerase Buffer (Invitrogen), 0.2 mM dNTPs mix, 1.5 mM MgCl 2 , 0.2 μM of each primer and 100 ng of gDNA. The following PCR reaction conditions were used: 95 °C for 2 min, 35 cycles of 95 °C denaturation for 30 s, 59 °C annealing for 30 s and 72 °C extension for 30 s, followed by a 5-min final extension at 72 °C. Matched non-tumoral surrounding tissues and in nine non-neoplastic liver tissues obtained from patients who underwent resection due to non-malignant liver conditions were analysed for the mutations. For IDH1/2 mutations screening, the PCR amplifications were performed in a volume of 25 μl reaction mixture containing 1.5 mM MgCl2, 0.2 mM of each dNTP, 0.125 mM of each primer and 1 U of Platinum Taq DNA Polymerase (Invitrogen). PCR products were purified using the Qiaquick PCR purification kit (Qiagen) and sequenced using an Applied Biosystems 3700 DNA sequencer (ABI PRISM 3730XL; Applied Biosystems). Immunoprecipitation and western blot analysis Proteins were extracted with RIPA buffer containing phosphatase (78428, ThermoScientific, Maltham, MA) and protease inhibitors (04693124001, Roche, Basel, Switzerland). Cell extracts were prepared from cells transiently or stably transfected with the mammalian expression empty vector or pDEST-V5-FGR2/PPHLN. The lysate (300 μg) was immunoprecipitated with anti-V5 antibody (1/250 dilution, cat#R960-25, Life Technology) for 3 h at 4C. Lysates were incubated with protein A/G Agarose beads (cat# 20423, Pierce) for 1 h at 4C. After the washing steps, beads were resuspended in Laemmli sample buffer. Immunoprecipitated V5-FGFR2–PPHLN1 fusion protein was detected by western blot using the anti-V5 antibody (1/1,000). Results were confirmed by using the anti-FGFR2 antibody (ab75984, Abcam, 1/1,000). Activation of V5-FGFR2–PPHLN1 was detected by western blot using the anti-phosphotyrosine clone 4G10 antibody (cat# 05-321, Millipore, 1/1,000). Thirty μg of proteins was loaded on 7.5–10% SDS gels and transferred to polyvinylidene difluoride membranes. Membranes were bovine serum albumin blocked and hybridized at 4 °C overnight with primary antibodies. Horseradish peroxidase-conjugated secondary antibody was applied at room temperature for 1 h. Blots were developed using RPN 2132 ECL plus solution (GE Healthcare) and imaged with FUJIfilm Laser Image Analyzer (GE Healthcare Life Sciences, Waukesha, WI). Antibodies against total ERK (#4695), MEK1/2 (#9122), ARAF (#4432) BRAF (#9433) phospho-ERK1/2(Thr202/Tyr204), (#9101), phosho-MEK1/2 (Ser217/Ser221) (#9121) were from Cell Signaling (Danvers, MA) and were used 1:2,000. Antibody against α-tubulin (T-5168) was from Sigma-Aldrich (St Louis, MO) and was used 1:2,000. Uncropped images have been provided and can be found in Supplementary Fig. 9 . Transforming activity of FGFR2–PPHLN1 and ARAF mutations Mouse NIH3T3 fibroblast cells were transfected with empty vector, FGFR2–PPHLN1 , ARAF WT, ARAF N217I, ARAF G322S. Colonies count was performed on day 21 using an inverted microscope. NIH3T3 cells transfected with FGFR2–PPHLN1 were cultured in the presence or absence of the FGFR inhibitor BGJ398 (1 μM). The compound solution was added to the top layer of soft agar every 3 days. In vitro functional assays Cells stably transfected with empty vector and destination vectors (3,000 per well) were plated in 96-well plates in triplicate. Cell proliferation was monitored after 24, 48 and 72 h using colorimetric 3-(4,5-dimethylthiazol-2yl)-5-(3-carboxymethoxyphenyl)-(4-sulfophenyl)-2H-tetrazolium assays (MTS; Promega) according to the manufacturer’s instructions. Optical densities were measured with a Biotek plate reader. Migration assay was performed using Transwell chambers (8-μmol l −1 pore size; BD Bioscience, Bedford, MA). In brief, 20,000 cells were resuspended in 250 μl of serum-free medium and plated in the upper chamber. Medium (650 μl) containing 5% fetal bovine serum was added to the lower chamber. Cells were incubated at 37 °C for ~24 h. After culture, cells that migrated from the upper well of a transwell chamber into the lower well were stained with crystal violet and counted [45] . For the clonogenic assay, cells were plated at low density (100 per well) in six-well plates in triplicates. Medium was changed twice per week. After 2 weeks, colonies were stained with crystal violet for 30 min and counted under a light microscope. The results are normalized to the control and presented as the mean of three independent experiments (mean+s.d.). Statistical significance was analysed by two-sided paired t -test. How to cite this article: Sia, D. et al . Massive parallel sequencing uncovers actionable FGFR2–PPHLN1 fusion and ARAF mutations in intrahepatic cholangiocarcinoma. Nat. Commun. 6:6087 doi: 10.1038/ncomms7087 (2015). Accession codes : The RNA sequencing and whole-exome sequencing data have been deposited in GEO under the accession code GSE63420 .